Observational constraints indicate risk of drying in the Amazon basin Climate warming due to human activities will be accompanied by hydrological cycle changes. Economies, societies and ecosystems in South America are vulnerable to such water resource changes. Hence, water resource impact assessments for South America, and corresponding adaptation and mitigation policies, have attracted increased attention. However, substantial uncertainties remain in the current water resource assessments that are based on multiple coupled Atmosphere Ocean General Circulation models. This uncertainty varies from significant wetting to catastrophic drying. By applying a statistical method, we characterized the uncertainty and identified global-scale metrics for measuring the reliability of water resource assessments in South America. Here, we show that, although the ensemble mean assessment suggested wetting across most of South America, the observational constraints indicate a higher probability of drying in the Amazon basin. Thus, over-reliance on the consensus of models can lead to inappropriate decision making. Combined with increasing water demand due to population growth and economic development, alterations in water availability due to climate change [1] , [2] will significantly impact human health, socioeconomic activities and ecosystems in South America [3] , [4] . Even in the present day, partly due to the lack of an adequate disaster prevention strategy, South American countries are vulnerable to floods and droughts related to unforced climate variability [3] . In addition, if water resources are scarce, the Amazon rainforest may be negatively affected, seriously impacting both biodiversity and the carbon cycle [5] , [6] , [7] . To inform adaptation and mitigation policies for future climate change, it is necessary to provide reliable water resource assessments. However, water resource assessments for South America are subject to substantial uncertainties [3] , [4] , [8] , [9] . As climate change projections from Atmosphere Ocean General Circulation models (AOGCMs) are fed into impact assessment models, AOGCM uncertainties also result in uncertain impact assessments [4] . Nevertheless, water resource impact studies (and other impact studies) have used projections from only a single or a few AOGCMs [4] for quite some time. Recently, impact studies have started to more vigorously incorporate projections from multiple AOGCMs [2] , [7] , [8] , [9] , [10] , [11] , [12] , [13] , [14] , [15] . However, studies regarding the mechanisms of the cascade of uncertainty and creditability in impact assessments are in their early stages. Multiple projections and/or impact assessments were used to create the best-estimate weighted ensemble mean (together with error bars) or the weighted ensemble distribution as an approximation of the probability density function. Whereas this paper focuses on the best estimate, the basic philosophy of weighting discussed below was used for both the best estimate and the probability density function. In the past, three primary approaches were used to weigh regional impact assessments from multiple AOGCMs. The first approach uses the equal-weighted ensemble, which has recently been called model democracy [16] . The creditability of an impact assessment is established by majority voting from AOGCMs based on the 'one-model, one-vote' assumption [9] , [11] , [12] , [14] , [15] . To move beyond this widely used, but naive, approach, the following two approaches have recently been investigated. One approach is to trust climate change projections from AOGCMs with high levels of accuracy for simulating the climate over a target region in the present [13] , [17] . However, because climate change patterns have spatial scales of several thousand to tens of thousands of kilometres, it is not clear whether regional climate simulations in the present can provide sufficient information for constraining the uncertainties. In the second approach, overall metrics of accuracy for global-scale present climate simulations (such as the root mean square error of the surface air temperature over a global domain) are used to select or weigh AOGCM projections in an attempt to reduce uncertainties of climate projections and relevant impact assessments. However, two studies using different overall metrics disagreed even about the sign of runoff changes in South America [8] , [10] . In addition, recent studies [18] , [19] have suggested that the association between overall metrics and future projections is weak in ensembles of AOGCMs. One intrinsic difficulty of establishing metrics for model skills and weights is that no observations of the future climate are available. Hence, we cannot evaluate the reliabilities of future projections by directly comparing them to any corresponding observations. Metrics should at least be physically reasonable and strongly related to future projections and impact assessments; however, there is no roadmap for determining adequate metrics [16] thus far. Here, we show how to identify global-scale metrics for measuring the reliability of runoff change assessments in South America. The observational constrains indicate a higher probability of drying in the Amazon basin than that expected by the model democracy approach. Uncertainty propagation There are substantial inconsistencies in annual mean runoff changes (Δ R ) in South America. Supplementary Figure S1 shows the pattern of Δ R from the observed climatology in 1980–1999 to the projected 2080–2099 mean under the A2 emissions scenario [20] for 14 AOGCMs ( Supplementary Table S1 ) and the ensemble mean. As in our previous study [2] , we performed ensembles of hydrological simulations using a global water resource model [21] (hereafter H08, see Methods) to obtain Δ R . Here, we did not take into account the uncertainties in the water resource models. The H08 inputs were the changes in temperature (Δ T ) and precipitation (percent change, Δ P ) from 14 AOGCMs. The Δ T , Δ P and Δ R were normalized by the global mean temperature change for each AOGCM, meaning that we did not take into account the uncertainty in the global mean temperature change. Whereas the ensemble mean assessment showed increases of Δ R over most areas of South America, the patterns of Δ R were remarkably different across models. We examined the physical mechanisms underlying uncertainty propagation from climate projections to Δ R ( Supplementary Fig. S2 ). We analysed the covariance matrix among 14 annual mean Δ R s in South America and 14 pairs of annual mean Δ T s and Δ P s over a global domain by applying singular value decomposition (SVD) analysis [22] , which has been used in meteorological studies (see Methods). This statistical method identifies pairs consisting of a Δ R mode and a (Δ T , Δ P ) mode ( Fig. 1a–d for the first mode and Fig. 1e–h for the second mode), so that the covariance between their expansion coefficients ( Supplementary Fig. S3 ) is maximized. The first Δ R mode shows a pattern of drying and wetting over the northern and southern areas of South America, respectively ( Fig. 1a ). This asymmetric pattern of Δ R in the north versus the south is related to an increase in Δ T over the eastern tropical Pacific Ocean ( Fig. 1b ), which is known as El-Niño-like warming [23] . AOGCMs with stronger El-Niño-like warming accompany a greater weakening of the Walker circulation ( Fig. 1d ). Downward and upward wind anomalies, which are atmospheric teleconnections of El-Niño-like warming, induce decreases and increases of Δ P in northern and southern South America, respectively ( Fig. 1c ). These changes in precipitation lead to the positive phase of the first Δ R mode. 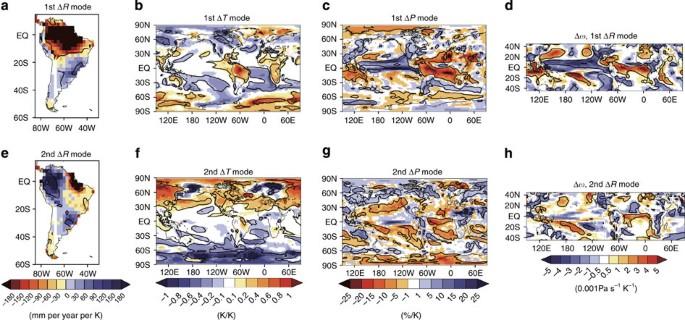Figure 1: First and second modes of the SVD analysis. (a) The first ΔRmode (mm per year per K). (b) The first ΔTmode (K/K). (c) The first ΔPmode (%/K). (d) The regression map between the expansion coefficient of the first ΔRmode and changes in vertical pressure velocity, averaged between 850 and 250 hPa (10−3Pa s−1K−1). (e) The second ΔRmode (mm per year per K). (f) The second ΔTmode (K/K). (g) The second ΔPmode (%/K). (h) The regression map between the expansion coefficient of the second ΔRmode and changes in vertical pressure velocity, averaged between 850 and 250 hPa (10−3Pa s−1K−1). Contours in the all panel indicate statistically significant correlations at ±10%t-test levels. Figure 1: First and second modes of the SVD analysis. ( a ) The first Δ R mode (mm per year per K). ( b ) The first Δ T mode (K/K). ( c ) The first Δ P mode (%/K). ( d ) The regression map between the expansion coefficient of the first Δ R mode and changes in vertical pressure velocity, averaged between 850 and 250 hPa (10− 3 Pa s −1 K −1 ). ( e ) The second Δ R mode (mm per year per K). ( f ) The second Δ T mode (K/K). ( g ) The second Δ P mode (%/K). ( h ) The regression map between the expansion coefficient of the second Δ R mode and changes in vertical pressure velocity, averaged between 850 and 250 hPa (10− 3 Pa s −1 K −1 ). Contours in the all panel indicate statistically significant correlations at ±10% t -test levels. Full size image The second Δ R mode shows drying over northeast South America and wetting over most of the other regions ( Fig. 1e ). This pattern of Δ R is related to positive and negative anomalies, relative to the ensemble mean, of Δ T over the Northern and Southern Hemispheres, respectively ( Fig. 1f ). This north–south gradient of Δ T is associated with a northward shift of the Hadley circulation [24] , [25] over the Atlantic Ocean ( Fig. 1h ). This shift of the Hadley circulation induced downward wind anomalies over northeast South America, resulting in decreases in the Δ P and Δ R values ( Fig. 1g,e ). Downward wind anomalies over northeast South America are related to a convergence of low-level horizontal winds over northwest South America, leading to upward wind anomalies ( Supplementary Fig. S4 ) and increases in Δ P and Δ R ( Fig. 1g,e ). The result, that Δ R in South America is influenced by El-Niño-like warming and the north–south Δ T gradient, is consistent with findings from previous studies [6] , [17] , [24] , [26] . Present climate patterns related to impact assessments Next, we investigated whether the leading Δ R modes were significantly correlated with particular, physically reasonable patterns of present climate simulations. 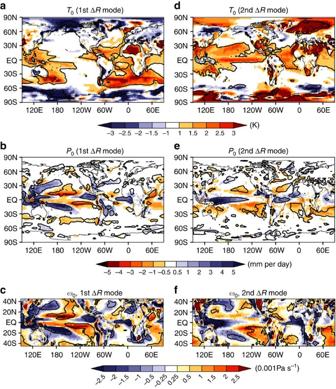Figure 2: Present climate patterns related to the runoff modes. (a) Regression maps betweenT0(K) in the present climate and the expansion coefficient of the first ΔRmode. (b) Regression maps betweenP0(mm per year) in the present climate and the first ΔRmode. (c) Regression maps between vertical pressure velocity, averaged between 850 and 250 hPa (10−3Pa s−1), in the present climate and the first ΔRmode. (d) Regression maps betweenT0(K) in the present climate and the expansion coefficient of the second ΔRmode. (e) Regression maps betweenP0(mm yr−1) in the present climate and the second ΔRmode. (f) Regression maps between vertical pressure velocity, averaged between 850 and 250 hPa (10−3Pa s−1), in the present climate and the second ΔRmode. Contours in the all panels indicate statistically significant correlations at ±10%t-test levels. Figure 2a–c shows the present climate (1980–1999) patterns of surface air temperature ( T 0 ), precipitation ( P 0 ) and atmospheric circulations regressed onto the expansion coefficients of the first Δ R mode in the impact assessments, respectively ( Supplementary Fig. S2 ). The first Δ R mode is correlated with a relatively warm T 0 over the tropical and subtropical ocean, but no significant correlation is found in the central tropical Pacific Ocean. This pattern of T 0 is associated with higher and lower P 0 values in the western and central tropical Pacific Ocean, respectively, and is related to stronger Walker circulations in the tropical Pacific Ocean. These results indicate that AOGCMs with a stronger Walker circulation in the present climate simulations ( Fig. 2c ) tend to have stronger El-Niño-like warming patterns in the future climate change projections ( Fig. 1b ), leading to a more positive phase for the first Δ R mode ( Fig. 1a ). Figure 2: Present climate patterns related to the runoff modes. ( a ) Regression maps between T 0 (K) in the present climate and the expansion coefficient of the first Δ R mode. ( b ) Regression maps between P 0 (mm per year) in the present climate and the first Δ R mode. ( c ) Regression maps between vertical pressure velocity, averaged between 850 and 250 hPa (10− 3 Pa s −1 ), in the present climate and the first Δ R mode. ( d ) Regression maps between T 0 (K) in the present climate and the expansion coefficient of the second Δ R mode. ( e ) Regression maps between P 0 (mm yr −1 ) in the present climate and the second Δ R mode. ( f ) Regression maps between vertical pressure velocity, averaged between 850 and 250 hPa (10− 3 Pa s −1 ), in the present climate and the second Δ R mode. Contours in the all panels indicate statistically significant correlations at ±10% t -test levels. Full size image Figure 2d–f shows the present climate patterns related to the second Δ R mode. The second Δ R mode is correlated with more intense precipitation in the Intertropical Convergence Zone of the Atlantic Ocean and a drier subtropical ocean in the present climate simulations. This intense Intertropical Convergence Zone accompanies stronger Hadley circulations over the Atlantic Ocean ( Fig. 2f ). AOGCMs with stronger Hadley circulations in the present climate simulations ( Fig. 2f ) tend to have larger northward shifts of the Hadley circulation in the future climate projections ( Fig. 1h ), leading to a more positive phase for the second Δ R mode ( Fig. 1e ). Despite considerable efforts of climate scientists, substantial uncertainties remain in the projections of El-Niño-like warming and the north–south Δ T gradient [23] , [27] , [28] . We identified relationships between future and present climate simulations that concern these phenomena. The physical mechanisms for the relationships between future and present climate simulations are not clear and remain to be investigated in future research. Global-scale metrics and observational constrains Here, to determine a set of metrics measuring bias magnitudes for each model corresponding to the leading Δ R modes, we computed the inner products of the vectors of bias patterns (the differences between the climatologies predicted by each model and actual observations) for each model ( Supplementary Figs S5 and S6 ) and the vectors of the present climate patterns associated with the leading Δ R modes ( Fig. 2 , the norms are normalized to 1; Supplementary Fig. S7 ). There are clear correlations between the expansion coefficients of the leading Δ R modes and the metrics of T 0 and P 0 (the value 0 indicates the best estimate; Fig. 3 ). An important finding is that the ensemble mean assessment of the runoff changes (with Δ R mode expansion coefficients of zero) has considerable negative biases for the present climate patterns corresponding to both the first and the second modes. Thus, we infer that the ensemble mean changes in the Walker and Hadley circulations are underestimated. This result is consistent with previous studies suggesting that past changes in the Walker and Hadley circulations of AOGCMs are smaller than those in the observations [28] , [29] , although it is not clear whether historical records are sufficient to constrain the model simulations [30] . 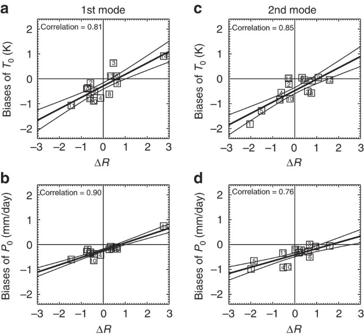Figure 3: Metrics for measuring the reliability of the runoff modes. (a) Scatter plot of the expansion coefficient of the first ΔRmode (normalized by the inter-model standard deviation) and theT0biases (K). (b) Scatter plot of the expansion coefficient of the first ΔRmode and theP0biases (mm per day). (c) Scatter plot of the expansion coefficient of the second ΔRmode and theT0biases (K). (d) Scatter plot of the expansion coefficient of the second ΔRmode and theP0biases (mm per day). The bold and thin lines indicate linear regressions and their corresponding 10 and 90%t-test-based confidence intervals, respectively. Figure 3: Metrics for measuring the reliability of the runoff modes. ( a ) Scatter plot of the expansion coefficient of the first Δ R mode (normalized by the inter-model standard deviation) and the T 0 biases (K). ( b ) Scatter plot of the expansion coefficient of the first Δ R mode and the P 0 biases (mm per day). ( c ) Scatter plot of the expansion coefficient of the second Δ R mode and the T 0 biases (K). ( d ) Scatter plot of the expansion coefficient of the second Δ R mode and the P 0 biases (mm per day). The bold and thin lines indicate linear regressions and their corresponding 10 and 90% t -test-based confidence intervals, respectively. Full size image In Figure 3 , about +0.7 and +1.6 s.d. of the first and second Δ R mode expansion coefficients (the intersections of the regression lines with the horizontal axes) yield the best estimate (the corresponding biases of the present climate simulations are zero). If we trust the equal-weighted ensemble mean assessment, then the best estimate is 'light wetting over most of South America' ( Fig. 4a ). By contrast, our evaluation based on the present climate observations suggests that 'drying over the Amazon basin and wetting over the La Plata basin and in northwestern South America' ( Fig. 4b ) is most plausible. 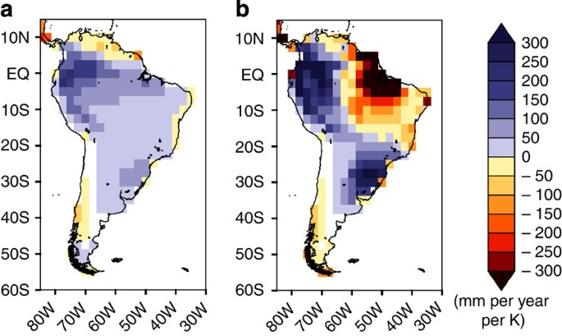Figure 4: The ensemble mean and best estimate of runoff changes. (a) Changes in runoff (mm per year per K) for the ensemble mean. (b) Changes in runoff (mm per year per K) for the observationally constrained best estimate. Figure 4: The ensemble mean and best estimate of runoff changes. ( a ) Changes in runoff (mm per year per K) for the ensemble mean. ( b ) Changes in runoff (mm per year per K) for the observationally constrained best estimate. Full size image In the Amazon basin, the sign of Δ R is different between the ensemble mean assessment and our observationally constrained assessment. Adaptation strategies used to cope with increases and decreases of runoff are very different. It has been suggested that an over-reliance on consensus assessments could lead to inappropriate adaptation policies relating to water resources. Notably, the observationally constrained assessment of Δ R seems qualitatively similar to that of the outlier model 14 (HadCM3; Fig. 4b and Supplementary Fig. S1 ), although this model overestimated the first Δ R mode ( Fig. 3a,b; also see Methods). This model projects catastrophic drying that could lead to dieback of the Amazon rainforest [5] , [6] . The probability of Amazon rainforest dieback could be higher than that indicated by projections based on model democracy. Recently, climate scientists have been actively exploring how to evaluate, beyond the use of model democracy, the reliability of climate change projections from AOGCMs [16] . Although there have been a few successful examples [31] , [32] , the problem is still significant [16] . By contrast, most impact assessment studies use the model democracy approach or the single-model approach. We stress that our study can be used as a possible roadmap for objective development of observational constraints on impact assessments and climate projections for a given target region. Our approach can be applied not only to water resource assessments but also to other impact assessments and climate projection studies. Investigations of the uncertainty of hydrological models remain for future work. It is better to use multiple global-scale hydrological models and the outputs from multiple AOGCMs. However, it is still difficult for us to use models developed by other institutes, although progress is being made in international coordinated intercomparison projects for global-scale hydrological models [33] . Although it will be possible to use multiple hydrological models in the future, we should advance our analysis methods so that we can investigate the uncertainty cascades from multiple AOGCMs to multiple hydrological models. The incorporation of the direct CO 2 effect on the transpiration of plants is a challenging issue for global-scale hydrological modelling and also remains to be investigated in future work. H08, along with most current hydrological models, does not take the CO 2 effect on plants into account. Some studies have suggested that the CO 2 effect on plants will have a major impact on future runoff [34] , [35] , whereas one study showed relatively small impacts [36] . An alternative methodological option is analysing the direct runoff outputs from the AOGCMs rather than the outputs of H08. AOGCMs have a variety of land hydrological schemes and some AOGCMs take the CO 2 effect on plants into account. However, runoffs from AOGCMs have considerable biases; for example, some AOGCMs have negative runoff values in their current climate simulations. The runoff biases in AOGCMs may be partly due to errors in land hydrological schemes and biases in the atmospheric hydrological cycles for the present climate. Therefore, it was preferable to use the outputs of H08 with bias corrections (see Methods) in this study. Hydrological simulations We computed Δ R using a global water resource model of H08 (refs 2 , 21 ) with a methodology typical of that adopted in previous studies of water resource assessments. H08 consists of six modules, including those for anthropogenic activities, but the two modules for natural hydrology (the land surface hydrology and the river routing modules) were used in this study. For the present climate simulation of runoff, we used the 1980–1999 meteorological forcing data set (NCC) [37] as the input data for H08. For future climate simulations of runoff, we altered the input data of H08 by adding Δ T to the NCC data and multiplying the NCC data by Δ P . It should be noted that these processes (adding Δ T to the NCC data and multiplying the NCC data by Δ P ) also act as simple bias correction techniques. By subtracting the runoff in the present climate from that in the future climate, we obtained 14 Δ R values. Grids with <1mm per month runoff were eliminated from the calculations. The spatial resolution of the outputs of H08 was 1°×1°, and those of the AOGCMs vary from model to model. For convenience of analysis, these data were interpolated to a 2.5°×2.5° regular latitude/longitude grid. If outputs of some ensemble members with different initial conditions were available for a given AOGCM ( Supplementary Table S1 ), we analysed their average. SVD analysis SVD analysis has often been used in meteorology [22] , [38] , but impact researchers may not be familiar with this methodology. Therefore, we describe the SVD method below. Here, M , N 1 and N 2 are the ensemble size (=14), the number of grids for Δ R and the number of grids for Δ T and Δ P , respectively. We define a i,k as Δ R for the k th model and i th grid: Vectors and are the Δ T and Δ P values of the k th model. is the combination of and : Here, we remove the ensemble means from and . We investigate the covariance matrix between A and B : Here, ( N 2 ×2)≥ N 1 . Before we compute C , the following preprocesses are applied. Because the units of Δ R , Δ T and Δ P are different from each other, we divide them by the corresponding inter-model standard deviations aggregated over the analysed areas. Furthermore, a i,k and b j,k are weighted by the square root of the cosine of the latitude. We compute the SVD of matrix C : Matrix ∑ is an N 1 × N 1 diagonal matrix with non-negative elements σ ll = σ l ( l =1,... N 1 ; , called singular values. Here and are the l th left and right singular vectors of C , respectively. The fraction of the squared Frobenius norm of the covariance matrix determined by the l th pair of the Δ R mode and the (Δ T , Δ P ) mode is computed by The first and second pairs explain about 45 and 20%, respectively, of the squared Frobenius norm ( Supplementary Fig. S3a ). The expansion coefficients of the Δ R mode ( ) and the (Δ T , Δ P ) mode ( ; Supplementary Fig. S3b–c ) are obtained by projecting A and B onto and , respectively: The correlation coefficient between the expansion coefficients, and , provides a measure of how strongly the Δ R mode and the (Δ T , Δ P ) mode are related to each other ( Supplementary Fig. S3d ). The first ten pairs have high correlations. By regressing A onto , we obtain the spatial pattern of Δ R corresponding to the l th (Δ T , Δ P ) mode: We also compute the spatial patterns of Δ T and Δ P corresponding to the l th Δ R mode by regressing B onto : These patterns are called heterogeneous regression maps. Figure 1a–c,e–g shows heterogeneous regression maps. Heterogeneous correlations are also computed using a similar procedure. We test the statistical significance of the heterogeneous correlations at ±10% t -test levels. Testing the influence of outlier model Our observationally constrained assessment of Δ R seems ro be similar to that of the outlier model 14 (HadCM3; Fig. 4b and Supplementary Fig. S1 ). It may be inferred that this single model had a dominant role in producing this result. However, as discussed below, our most plausible Δ R pattern changed little when we excluded HadCM3 from our analyses. We tested whether our most plausible Δ R pattern is sensitive to the exclusion of HadCM3 from our analyses. Although the first and second modes of Δ R and (Δ T , Δ P ) obtained using the 13 AOGCMs ( Supplementary Fig. S8 ) were similar to those of all of the 14 AOGCMs ( Fig. 1 ), there were some differences. Here, we defined and as the spatial pattern vectors of the first and second Δ R modes, respectively, using all 14 AOGCMs ( Fig. 1 ). In addition, and were the first and second runoff modes when we excluded HadCM3 from our analyses ( Supplementary Fig. S8 ). When we projected and onto and (before the projections, their norms were normalized to 1), it appeared that and were mixtures of and : Thus, the present climate patterns associated with and ( Supplementary Fig. S9 ) were also somewhat different from those of and ( Fig. 2 ). The most plausible and modes were about −0.5 and +1.6 s.d. of their expansion coefficients, respectively ( Supplementary Fig. S10 ). Supplementary Figure S11 demonstrates the runoff changes in the ensemble mean and the best estimate. Although the drying region in the Amazon basin is narrower in the Supplementary Figure 11b than in Figure 4b , these patterns are qualitatively similar to each other. Therefore, our estimates of the most plausible Δ R patterns are not sensitive to the inclusion of HadCM3 in our analyses. Testing the influence of internal variability Here, we tested whether our finding is sensitive to the influence of internal variability. For some models, the outputs from members of different initial condition ensembles (DICEs) were available ( Supplementary Table S1 ). In this case, to reduce the influence of internal variability on our results, we used the average of the DICE members for each model in our analyses. Here, we computed the first and second Δ R mode coefficients and the corresponding T 0 and P 0 biases for each DICE member ( Supplementary Fig. S12 ). There is little difference between the DICE members for each model. Therefore, our finding is not sensitive to the influence of internal variability. How to cite this article: Shiogama, H. et al . Observational constraints indicate risk of drying in the Amazon basin. Nat. Commun. 2:253 doi: 10.1038/ncomms1252 (2011).